Identification and characterization of polyclonal αβ-T cells with dendritic cell properties An efficient immune response requires coordination between innate and adaptive immunity, which act through cells different in origin and function. Here we report the identification of thymus-derived αβ-T-cell receptor + cells that express CD11c and major histocompatibility complex class II, and require FLT3 ligand for development (T DC ). T DC express genes heretofore found uniquely in T cells or dendritic cells, as well as a distinctive signature of cytotoxicity-related genes. Unlike other innate T-cell subsets, T DC have a polyclonal T-cell receptor repertoire and respond to cognate antigens. However, they differ from conventional T cells in that they do not require help from antigen-presenting cells, respond to Toll-like receptor-mediated stimulation by producing interleukin-12 and process and present antigen. The physiological relevance of T DC , found in mice and humans, is still under investigation, but the fact that they combine key features of T and dendritic cells suggests that they provide a bridge between the innate and adaptive immune systems. An efficient immune response requires coordination between innate and adaptive immunity [1] . In particular, crosstalk between dendritic cells (DCs) and T cells is key in the initiation of adaptive immunity [2] , and both of those cell types are thought to have clearly distinct roles during this process. DCs, the most efficient antigen-presenting cells (APCs), process and present pathogen-associated antigens in the form of peptides loaded on major histocompatibility complex (MHC) molecules. The course of a particular adaptive immune response is shaped by the maturation and activation status of DCs, with immature DCs leading to tolerance and mature DCs to efficient immune responses. One way DCs are induced to mature is ligation of pattern-recognition receptors by specific microbial-associated patterns [3] , which results in upregulation of costimulatory molecules and MHC-II, as well as production of pro-inflammatory cytokines such as IL-12 and tumour necrosis factor-α. On maturation, DCs migrate to T-cell areas in the peripheral lymphoid organs, where they present antigen loaded on MHC-II molecules to CD4 + T cells. Some DCs are also very efficient in cross-presentation of viral or endogenous peptides on MHC-I molecules to CD8 + T cells. Recognition of MHC complexes by the T-cell receptor (TCR) combined with costimulation provided by mature DCs results in a complete and effective adaptive T-cell response [2] . Although both arise from bone marrow progenitors, the developmental paths of DCs and T cells diverge early and are thought to be as distinct as their functions. Conventional DCs (cDCs) originate from a common DC progenitor in the bone marrow and migrate to peripheral lymphoid organs [4] . Transcription factors such as PU.1, Ikaros, IRF8, RelB and Batf 3 have been implicated in DC development, but due to their pleiotropic role and the high heterogeneity of DC subsets none of these can be used to exclusively define the DC lineage [5] , [6] . Two recent papers reported that the transcription factor Zbtb46 is expressed by cDCs throughout their differentiation, and is a specific marker for cDCs among immune cells [7] , [8] . Although no master regulator of DC lineage commitment has been described, interactions of FLT3 with its ligand (FLT3L) are necessary for DC development and homeostasis, because FLT3L-deficient mice lack DCs in peripheral lymphoid organs [9] . In contrast to DCs, T-cell commitment occurs in the thymus, where T-cell precursors undergo a multi-step process that leads to the generation of mature CD4 + CD8 − and CD4 − CD8 + T cells [10] , [11] . The most immature thymocytes are CD4 − CD8 − (double negative (DN)) and can be separated into four different populations (DN1–4) based on expression of CD44 and CD25. DN1–DN2 thymocytes retain the plasticity to give rise to some myeloid cell types, including natural killer (NK) cells and thymic DCs [11] , [12] , [13] , [14] . Commitment to the T-cell lineage, and the subsequent recombination of the TCRβ locus and pre-TCR expression, takes place at the DN3 stage (CD25 + CD44 − ), is Notch-dependent, and subsequent to the silencing of a number of transcription factors important for myeloid development, most notably PU.1 [14] . Although innate and adaptive immune systems have been thought to act through different cells and mechanisms, recent studies provide several examples in which these two arms of the immune system appear to overlap. For example, some thymus-selected T cells, such as NK T cells [15] and most γδ-T cells [16] , are considered innate because of their limited TCR repertoire and prompt responses to non-peptide antigens. There is also evidence that some T cells can express low but detectable levels of Toll-like receptors (TLRs) [17] , which are normally involved in maturation and activation of DCs and other innate immune cells [3] . However, the outcome of TLR triggering in T cells is different from that in innate immune cells, being confined to increased survival and costimulation [17] , [18] . These observations prompted us to ask whether there exist cells that truly combine the molecular and functional characteristics of innate and adaptive immunity. We have identified a novel population of thymus-derived cells that, like DCs, require FLT3L for development and exhibit surface markers and functions of both DC and T cells (T DC ). Molecular profiling revealed that T DC express genes characteristic of DCs, T cells and cytotoxic cells. T DC expressed polyclonal αβ-TCRs and responded to antigen, but unlike conventional T cells did not require help from APCs. Strikingly, T DC responded to TLR-mediated stimulation by producing IL-12, and were able to process and present antigen to MHC-II-restricted T cells. Identification of cells expressing DCs and T-cell markers Conventional murine DCs express high levels of CD11c and MHC-II. Interestingly, we found that around 7% of splenic DCs expressed αβ-TCR, a distinguishing characteristic of conventional αβ-T cells ( Fig. 1a ). These cells comprised 0.04% of spleen and 0.06% of lymph node cells ( Fig. 1b ), and because they expressed T-cell and DC, but not other lineage markers ( Fig. 1c ), were termed T DC . T DC were positive for T-cell markers such as Thy-1, CD27, and either CD4 or CD8β at the same ratio as conventional T cells ( Fig. 1d ). T DC had a polyclonal Vβ repertoire comparable to conventional αβ-T cells ( Fig. 1f ), in marked contrast to previously described semi-invariant innate T-cell subsets [15] . As CD11c can be expressed on activated T cells in some infectious settings [19] , [20] , [21] , we asked whether T DC might represent a subset of activated T cells. T DC displayed neither signs of recent activation (CD69 − CD25 − IL-7R hi ) nor showed an increase in T-cell memory markers CD122 or CXCR3 ( Fig. 1g ). The homing molecules CCR7 and CD62L were expressed similarly in T cells and T DC , but not in DCs. In fact, expression levels of all of the tested T-cell markers on T DC mirrored the levels on T cells. One activation/memory T-cell marker, CD44, was expressed on T DC , but was expressed equally on DCs, and thus in this case cannot be considered a T-cell marker. Staining for DC markers revealed that T DC expressed CD11c, MHC-II, CD11b, F4/80 and FcRγ at intermediate levels with respect to cDCs ( Fig. 1h and Supplementary Fig. 1a ) whereas non-DC-specific markers such as MHC-I and CD45 were expressed at similar levels ( Supplementary Fig. 1a ). To test whether T DC are T cells that acquired DC markers through intercellular transfer [22] , cells from a reporter mouse that reveal transcriptional regulation of CD11c were examined. Just as with cell surface CD11c ( Fig. 1h ), T DC enhanced green fluorescent protein (EGFP) expression driven by the CD11c promoter was at levels intermediate between T cells and DCs ( Fig. 2a and Supplementary Fig. 1b ). Furthermore, highly purified ( Supplementary Fig. 1c ) T DC expressed Ciita , which regulates transcription of MHC-II and is not expressed by murine T cells [23] ( Fig. 2b ). In the obverse approach, a GFP reporter driven by the Thpok-regulatory elements, a transcription factor active in CD4 T cells [24] , was expressed in CD4 + but not CD8 + T DC ( Fig. 2c ). Therefore, expression of cell surface T and DC markers in T DC is a reflection of their transcriptional regulation. 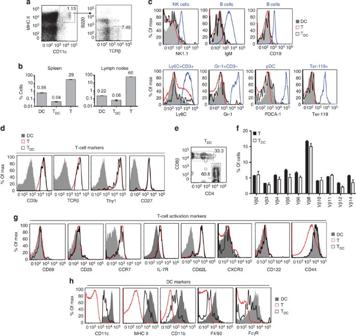Figure 1: Identification of murine cells expressing T-cell and DC markers (TDC). (a) Gating strategy for identification of TDCfrom B6 splenocytes. (b) The frequencies of the indicated subsets are shown in spleen and lymph nodes of at least 10 B6 mice. Mean±s.e.m. is represented for each cell subset. (c–h) Surface marker expression by the indicated subsets from B6 splenocytes. (f) Mean±s.e.m. of three mice is represented for each marker. Figure 1: Identification of murine cells expressing T-cell and DC markers (T DC ). ( a ) Gating strategy for identification of T DC from B6 splenocytes. ( b ) The frequencies of the indicated subsets are shown in spleen and lymph nodes of at least 10 B6 mice. Mean±s.e.m. is represented for each cell subset. ( c – h ) Surface marker expression by the indicated subsets from B6 splenocytes. ( f ) Mean±s.e.m. of three mice is represented for each marker. 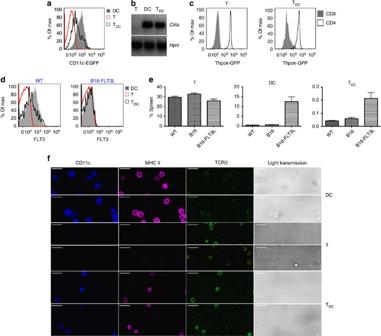Figure 2: TDCare single cells expressing T and DC molecules and expand in response to FLT3L. (a,c) Fluorescence reporter expression in splenocytes of CD11c-EGFP (a) or Thpok-GFP (c) reporter mice. (b) RT–PCR analysis of double-sorted cell subsets from B6 splenocytes. (d,e) B6 mice were injected subcutaneously in the back with B16 or B16-FLT3L melanoma cells. Ten to thirteen days after injection the indicated splenocyte subsets were analyzed for surface FLT3 levels (d) or frequency (e). The mean±s.e.m. of each subset from 2 (B16-injected) or 10 mice (wild type (WT) or B16-FLT3L) is shown in (e). Cells from uninjected mice are shown as a control (WT). (f) Confocal microscopy analysis of cells from double-sorted splenocytes of B16-FLT3L-injected mice. Scale bars, 20 μm. One representative experiment of at least three is shown in each panel. Full size image Figure 2: T DC are single cells expressing T and DC molecules and expand in response to FLT3L. ( a , c ) Fluorescence reporter expression in splenocytes of CD11c-EGFP ( a ) or Thpok-GFP ( c ) reporter mice. ( b ) RT–PCR analysis of double-sorted cell subsets from B6 splenocytes. ( d , e ) B6 mice were injected subcutaneously in the back with B16 or B16-FLT3L melanoma cells. Ten to thirteen days after injection the indicated splenocyte subsets were analyzed for surface FLT3 levels ( d ) or frequency ( e ). The mean±s.e.m. of each subset from 2 (B16-injected) or 10 mice (wild type (WT) or B16-FLT3L) is shown in ( e ). Cells from uninjected mice are shown as a control (WT). ( f ) Confocal microscopy analysis of cells from double-sorted splenocytes of B16-FLT3L-injected mice. Scale bars, 20 μm. One representative experiment of at least three is shown in each panel. Full size image FLT3L is a hematopoietic growth factor often used to expand DCs in vivo [25] . To test whether T DC resemble DCs in this regard, after assessing that T DC express FLT3 ( Fig. 2d , left), C57BL/6 (B6) mice were injected with B16-FLT3L melanoma cells. As described for cDCs [25] , [26] , T DC downregulated FLT3 ( Fig. 2d , right) and expanded in response to FLT3L, resulting in a five to sixfold increase in frequency ( Fig. 2e ). FLT3L-expanded T DC had a cell surface phenotype identical to T DC in unmanipulated mice (data not shown), and were used in experiments when indicated. We considered the possibility that T DC represented rare T-cell/DC doublets that escaped doublet discrimination detection ( Supplementary Fig. 1d ). Arguing against this was that the levels of the T-cell markers on T DC were indistinguishable from conventional αβ-T cells, whereas DC markers were intermediate between T cells and DCs. Moreover, a radiation bone marrow chimera showed that each newly generated T DC displayed only one of the two congenic markers, never both, indicating that they are not T/DC conjugates ( Supplementary Fig. 1e ). Perhaps the best evidence came from imaging highly purified T DC by confocal microscopy ( Fig. 2f ). Whereas T cells were TCR + CD11c − MHC-II − and DCs were TCR − CD11c + MHC-II + , each T DC bore all three markers. T DC size and morphology was similar to T cells, not DCs, suggesting that they are a novel subset of T cells with innate cell characteristics. T DC have a unique gene signature cDNA microarray analyses were performed to provide a non-biased assessment of T DC gene expression, and revealed that T DC have a clearly distinct genetic profile ( Fig. 3a ). T DC expressed many genes encoding proteins normally found in T cells (for example, Lck, CD3 subunits and IL-7Rα) or DCs (CD83, MHC-II, FLT3 and Zbtb46), but not both ( Tables 1 and 2 ). Many of the cell surface proteins identified by microarray were among those detected on T DC in Fig. 1 . In addition, T DC expressed Itgal (encoding CD11a, the α chain of the integrin LFA-1, which is upregulated in activated T cells) at levels comparable to those of DCs and unstimulated T cells (data not shown). PU-1 (encoded by Sfpi1 ) is a myeloid lineage-related transcription factor [5] , and Zbtb46 has recently been shown to be expressed specifically in DCs [7] , [8] . Their expression in T DC and DCs but not T cells was validated by reverse transcription (RT)–PCR ( Fig. 3b ). Interestingly, some T DC -associated genes were expressed at much higher levels than in T cells or DCs. Among these were genes encoding granzymes A and B and eomesodermin, proteins normally expressed in cytotoxic cells, such as NK and effector CD8 + T cells. The relatively high expression of these genes in T DC was confirmed by RT–PCR, which revealed that Gzma was detectable only in T DC , whereas Gzmb and Eomes were expressed in T cells but at lower levels than in T DC ( Fig. 3b ). Similar results were obtained with RT–PCR for Prf1 , which encodes cytotoxic molecule perforin. Intracellular staining revealed that ~20% of CD8 + T DC expressed granzyme B in the absence of stimulation, whereas although a small amount of mRNA was found by RT–PCR ( Fig. 3b ), the protein was undetectable in T cells ( Fig. 3c ). Therefore, in addition to sharing characteristics with T cells and DCs, T DC exhibited a distinct molecular profile exemplified by cytotoxic gene expression. It is notable that T DC express a cytotoxic signature without signs of activation ( Fig. 1g ). 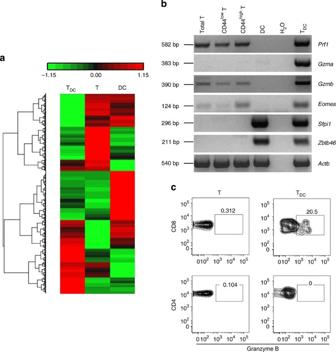Figure 3: Molecular profiling of TDCreveals a distinct genetic signature. (a) Gene expression heat map from microarray analysis of highly purified cells pooled from 12 B6 mice. Individual cell subsets are represented as columns. (b) RT–PCR of highly purified cells pooled from five B6 mice. One representative experiment of two to four independent analyses is shown. (c) Flow cytometric analysis of intracellular granzyme B in splenic T or TDCfrom B6 mice. Figure 3: Molecular profiling of T DC reveals a distinct genetic signature. ( a ) Gene expression heat map from microarray analysis of highly purified cells pooled from 12 B6 mice. Individual cell subsets are represented as columns. ( b ) RT–PCR of highly purified cells pooled from five B6 mice. One representative experiment of two to four independent analyses is shown. ( c ) Flow cytometric analysis of intracellular granzyme B in splenic T or T DC from B6 mice. Full size image Table 1 Selected genes expressed by T DC and DCs represented as fold difference with respect to T cells. Full size table Table 2 Selected genes expressed by T DC and T cells represented as fold-difference with respect DCs. Full size table T DC require a thymus and positive selection for development Conventional αβ-T cells require the thymus for development. Consistent with a similar requirement for T DC , bone marrow cell cultures supplemented with granulocyte–monocyte-colony-stimulating factor or FLT3L did not give rise to T DC (data not shown). In the thymus, a small percentage of cells expressing CD11c and MHC-II was found within both the CD3 int and CD3 hi subsets ( Fig. 4a ). A requirement for T DC development in the thymus was confirmed by the observation that T DC were not detected in the spleens of athymic nude mice ( Fig. 4b ). To determine whether T DC , such as αβ-T cells, undergo antigen-specific selection in the thymus, mice expressing αβ-TCR transgenes (Tg) on either positively selecting or non-selecting MHC haplotypes were studied. Rag2 −/− AND TCR Tg thymocytes are positively selected on H-2 b and H-2 k , but not the H-2 q haplotype [27] , [28] . T and T DC were present in mice with positively selecting haplotypes but not in mice of the non-selecting MHC, strongly suggesting that T DC require the same thymic-positive selection signals as conventional T cells ( Fig. 4c ). Additional evidence that T DC undergo positive selection came from studies of T DC Thpok expression, a transcription factor essential for CD4 expression in mature T cells. As seen in conventional T cells [24] , Thpok −/− mice lacked CD4 + T DC , and CD8 + T DC frequency was increased ( Fig. 4d ). To formally demonstrate that CD4 lineage-selected T DC were not lost but redirected to the CD8 lineage, a GFP reporter that monitors Thpok promoter activity was used in Thpok-deficient mice [24] to allow detection of CD4 lineage-selected T DC (CD8 + GFP + ) within the CD8 + T DC population ( Fig. 4e ). Together, these findings demonstrate that T DC are similar to conventional T cells in their origin and development. 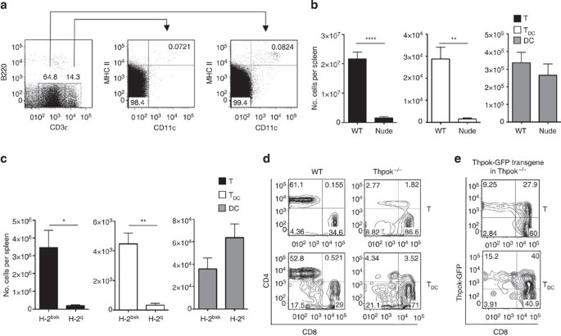Figure 4: TDCneed a thymus and positive selection for development. (a) Gating strategy for identification of TDCin B6 thymocytes. (b,c) Absolute numbers of the indicated cell subsets in spleens of athymic nude mice (b) or AND TCR Tg mice on H-2bxkor H-2qMHC haplotypes (c). Mean±s.e.m. of at least four mice per group, statistical analysis performed with a two-tailed Student’st-test. *P<0.05, **P<0.01, ****P<0.001. (d,e) Splenocytes of B6 wild-type (WT), Thpok−/−(d) or Thpok−/−-Thpok-GFP mice (e) were analyzed for CD4, CD8 and GFP expression. Figure 4: T DC need a thymus and positive selection for development. ( a ) Gating strategy for identification of T DC in B6 thymocytes. ( b , c ) Absolute numbers of the indicated cell subsets in spleens of athymic nude mice ( b ) or AND TCR Tg mice on H-2 bxk or H-2 q MHC haplotypes ( c ). Mean±s.e.m. of at least four mice per group, statistical analysis performed with a two-tailed Student’s t -test. * P <0.05, ** P <0.01, **** P <0.001. ( d , e ) Splenocytes of B6 wild-type (WT), Thpok −/− ( d ) or Thpok −/− -Thpok-GFP mice ( e ) were analyzed for CD4, CD8 and GFP expression. Full size image T DC have T-cell functional properties The ability of T DC to respond to TCR-mediated stimulation was assessed by stimulating splenocytes with anti-CD3. After stimulation, T DC displayed high levels of the activation marker CD69 ( Fig. 5a ). TCR-mediated T-cell proliferation requires stimulation via costimulatory receptors whose ligands are provided by APCs such as DCs [29] . Furthermore, stimulation with soluble anti-CD3 antibodies requires their immobilization by APC Fc receptors. As T DC exhibit DC characteristics and expressed CD80/CD86 ( Supplementary Fig. 2a ), we hypothesized that they might be able to provide these necessary functions for themselves. To test this, highly purified T cells or T DC were stimulated with soluble anti-CD3. In contrast to T cells alone, T DC expanded, and to a greater extent than T cells cocultured with DCs ( Fig. 5b ), indicating that they do not need help from conventional APC. Interestingly, whereas T DC activated via the TCR for up to 20 h retained their DC markers (data not shown), they lost them after proliferating ( Supplementary Fig. 2b ). To address the possibility that this might be due to expansion of a very small number of contaminating conventional T cells, we crossed Rosa26-YFP mice, which express fluorescent YFP only if a stop codon between the Rosa26 promoter and YFP is excised by Cre [30] , with CD11c-Cre-expressing animals. YFP expression was observed in the majority of DCs and T DC , and YFP bright cells were isolated by sorting ( Supplementary Fig. 2c ) and stimulated with soluble anti-CD3 ( Fig. 5c ). T DC expanded in culture and lost cell surface CD11c but maintained YFP expression. Importantly, YFP was not acquired by conventional T cells expanded in the presence of DCs. Thus, T DC expand in response to TCR-mediated stimulation. The question of whether T DC respond to cognate antigen was addressed with αβ-TCR Tg mice, all of which that we examined had T DC ( Supplementary Fig. 2d ). T DC sorted from OTII-Tg mice and stimulated with cognate antigen (chicken ovalbumin (OVA) peptide 323–329) proliferated in the absence of any additional APC, whereas conventional T cells did not ( Fig. 5d ). Thus, T DC have a functional TCR and are self-sufficient for antigen presentation. 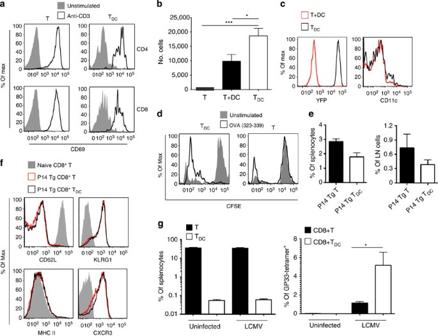Figure 5: TDChave T-cell functional properties. (a) Upregulation of CD69 on B6 splenocytes stimulated with soluble anti-CD3 for 18 h. (b,c) Cell counts and YFP expression of TDCor T cells double-sorted from B6 (b) or Rosa26-CD11c-Cre-YFP (c) splenocytes, stimulated with soluble anti-CD3, supplemented with IL-2 on day 3 and analyzed on day 8. Mean±s.e.m. of four independent experiments is shown in (b). (d) Carboxyfluorescein diacetate succinimidyl ester (CFSE) dilution of double-sorted TDCor T cells from OTII-Tg mice and stimulated with OVA 323–339 peptide (6.7 μM) for 7 days. (e) Frequency and surface markers (f) of double-sorted P14 TCR Tg TDCor T cells adoptively transferred at a 1:1 ratio into B6 mice, infected the next day with LCMV Armstrong and analysed 8 days later. Mean±s.e.m. of three independent experiments is shown in (e,g). Frequency of the indicated cell subsets from B6 mice infected with LCMV Armstrong strain 2 months earlier. Mean±s.e.m. of six mice is shown, and a two-tailed Student’st-test was performed. *P<0.05, ***P<0.005. Figure 5: T DC have T-cell functional properties. ( a ) Upregulation of CD69 on B6 splenocytes stimulated with soluble anti-CD3 for 18 h. ( b , c ) Cell counts and YFP expression of T DC or T cells double-sorted from B6 ( b ) or Rosa26-CD11c-Cre-YFP ( c ) splenocytes, stimulated with soluble anti-CD3, supplemented with IL-2 on day 3 and analyzed on day 8. Mean±s.e.m. of four independent experiments is shown in ( b ). ( d ) Carboxyfluorescein diacetate succinimidyl ester (CFSE) dilution of double-sorted T DC or T cells from OTII-Tg mice and stimulated with OVA 323–339 peptide (6.7 μM) for 7 days. ( e ) Frequency and surface markers ( f ) of double-sorted P14 TCR Tg T DC or T cells adoptively transferred at a 1:1 ratio into B6 mice, infected the next day with LCMV Armstrong and analysed 8 days later. Mean±s.e.m. of three independent experiments is shown in ( e , g ). Frequency of the indicated cell subsets from B6 mice infected with LCMV Armstrong strain 2 months earlier. Mean±s.e.m. of six mice is shown, and a two-tailed Student’s t -test was performed. * P <0.05, *** P <0.005. Full size image To assess T DC responses in vivo , equal numbers of lymphocytic choriomeningitis virus (LCMV) glycoprotein (gp)33–41-specific P14 Tg T DC and conventional T cells were adoptively transferred into wild-type hosts, which were then infected with LCMV. T DC and T-cell expansion was similar at day 8, the peak of the response ( Fig. 5e ). Moreover, comparable to the transferred T cells, all T DC had an activated phenotype: CD62L lo , KLRG1 hi and CXCR3 hi ( Fig. 5f ). Interestingly, T DC lost expression of MHC-II, acquiring a conventional T-cell phenotype after LCMV-mediated expansion, as had been seen after proliferation in vitro . Analysis 2 months after LCMV infection, when numbers of both T and T DC are at steady-state levels ( Fig. 5g , left), found gp33 tetramer + , and therefore antigen-experienced, T DC that presumably had re-acquired MHC-II ( Fig. 5g , right). Notably, a relatively high percentage of T DC were gp33-tetramer-positive, indicating that memory T DC persist in vivo like conventional memory T cells. T DC respond to TLR agonists in a DC-like manner The innate characteristics of T DC were explored. Unlike T cells, DCs require signaling via FLT3 for development and maintenance [9] . Notably, the fraction of T DC was markedly reduced in mice lacking the ligand for FLT3, FLT3L, to an extent similar to DCs ( Fig. 6a ). To test the ability of T DC to respond like innate immune cells, total splenocytes were stimulated with lipopolysaccharide (LPS) ( Fig. 6b ) or other TLR agonists ( Supplementary Fig. 3a ). T DC upregulated costimulatory molecules in a manner remarkably similar to DCs ( Fig. 6b ), whereas no upregulation was observed for conventional T cells (data not shown). In addition, T DC stimulated with TLR agonists produced IL-12, a cytokine produced by DCs and important for Th1 polarization ( Supplementary Fig. 3b ). IL-12 production by T DC was even more notable when splenocytes were primed with recombinant interferon-γ (rIFN-γ) followed by LPS stimulation ( Fig. 6c ). A prominent characteristic of DCs is their ability to process and present antigens on MHC-II. Purified T DC or DCs were co-cultured with OTII Tg T cells in the presence of whole-OVA protein. T DC -induced antigen-specific T-cell proliferation similar to DCs ( Fig. 6e ), indicating that T DC can process as well as present antigen on MHC-II. Thus, T DC have functional properties characteristic of bona fide innate cells. 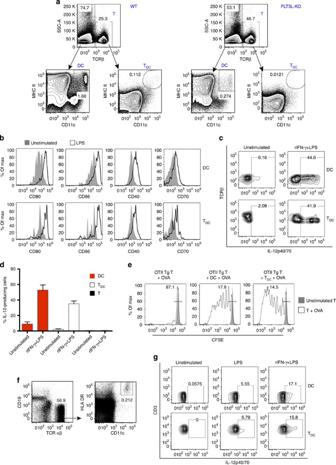Figure 6: TDChave DC properties and can be detected in human blood. (a) The indicated cell subsets from wild-type (WT) and FLT3L-deficient mice were stained and analyzed. One representative experiment of two is shown. (b) Flow cytometric analysis of surface costimulatory molecules in B6-gated splenic TDCstimulated with LPS (100 ng ml−1) for 24 h. (c–d) Representative experiment (c) or mean±s.e.m. of three mice (d) depicting IL-12 production by splenocytes of B6 mice primed with rIFN-γ (50 ng ml−1) and stimulated with LPS (200 ng ml−1) for 18 h. (e) Carboxyfluorescein diacetate succinimidyl ester (CFSE) dilution in >99% pure OTII Tg T cells co-cultured with double-sorted TDCor DCs stimulated with whole-OVA protein (50 μg ml−1). (f) Gating strategy for identification of TDCfrom human peripheral blood mononuclear cells. (g) Intracellular IL-12 production by human TDCstimulated with LPS (200 ng ml−1) for 24 h in the presence or absence of recombinant rIFN-γ (50 ng ml−1). One representative experiment of three is shown. Figure 6: T DC have DC properties and can be detected in human blood. ( a ) The indicated cell subsets from wild-type (WT) and FLT3L-deficient mice were stained and analyzed. One representative experiment of two is shown. ( b ) Flow cytometric analysis of surface costimulatory molecules in B6-gated splenic T DC stimulated with LPS (100 ng ml −1 ) for 24 h. ( c – d ) Representative experiment ( c ) or mean±s.e.m. of three mice ( d ) depicting IL-12 production by splenocytes of B6 mice primed with rIFN-γ (50 ng ml −1 ) and stimulated with LPS (200 ng ml −1 ) for 18 h. ( e ) Carboxyfluorescein diacetate succinimidyl ester (CFSE) dilution in >99% pure OTII Tg T cells co-cultured with double-sorted T DC or DCs stimulated with whole-OVA protein (50 μg ml −1 ). ( f ) Gating strategy for identification of T DC from human peripheral blood mononuclear cells. ( g ) Intracellular IL-12 production by human T DC stimulated with LPS (200 ng ml −1 ) for 24 h in the presence or absence of recombinant rIFN-γ (50 ng ml −1 ). One representative experiment of three is shown. Full size image To determine whether T DC exist in humans, peripheral blood lymphocytes from uninfected donors were analyzed. Approximately 0.2% of CD3 + TCRαβ + cells were positive for CD11c and human leukocyte antigen-DR (MHC-II), but unlike murine T DC the levels of these molecules were similar to those on cDCs ( Fig. 6f and Supplementary Fig. 3c ). Human T DC expressed T-cell markers at the same levels as conventional T cells, and like their murine counterparts, were single positive for CD4 or CD8 ( Supplementary Fig. 3d ). As activated human CD4 + T cells expressing MHC-II have been described [31] , we asked whether human T DC behave like innate immune cells. Human T DC stimulated with LPS produced IL-12 ( Fig. 6g ). Treatment with rIFN-γ before LPS stimulation increased IL-12 production by T DC , as it did for DCs. Here, we report the identification of T DC , a subset of cells characterized by the coexistence of features of conventional polyclonal T cells and DCs. Similar to another rare but notable DC subset, plasmacytoid DC, T DC have lymphocyte-like rather than DC morphology and express intermediate levels of CD11c and MHC-II (ref. 32 ). The fact that T DC recombine and express a functional TCR, but also have the ability to respond to TLR stimuli in a rapid, DC-like manner places T DC in the heterogeneous category of ‘innate T cells’. However, T DC substantially differ from other innate T cells primarily due to antigen-specific selection processes indistinguishable from classical αβ cells and the ability to mount a full-scale proliferative response to cognate antigens, both of which are essential in adaptive immunity. Moreover, they are negative for CD122, CD69 and CD25, markers constitutively expressed by NKT cells, and do not express NK lineage markers such as NK1.1 (refs 16 , 33 , 34 ). It is generally thought that cDCs and T cells originate from different precursors and pursue unrelated developmental programs [4] , [11] . The identification of T DC , which express lineage-specific markers of both DCs (PU.1 and Zbtb46) and T cells (TCR αβ), suggests that the lymphoid and myeloid differentiation pathways are not mutually exclusive, as previously thought. Whereas DN2 thymocytes, before T-cell commitment, retain the potential to generate both myeloid and NK progeny [14] , a mature cell seemingly committed to both T and DC lineages, with the capacity to respond in either a T- or DC-like manner, has not been described. If anything, myeloid and T-cell commitment are generally thought to be mutually exclusive. For example, forced expression of PU.1 at the DN3 stage inhibits T-cell development, strongly arguing for its role in terminating T-cell lineage commitment [35] . It is noteworthy, however, that signaling through Notch, initially thought to exclusively promote T-cell lineage commitment, can also promote the development of Thy1 + DCs in bone marrow cultures [36] and the differentiation of some DC subsets in the periphery [37] . Such findings could perhaps explain how some cell types might escape what was thought to be a rule for T-cell lineage commitment. cDNA microarray analysis revealed that T DC expressed a number of genes that were not found in DCs or T cells. This distinct genetic profile identifies them as a separate cell type and raises the possibility that T DC may have functions other than those of these two cell types. In particular, T DC express granzymes and perforin at very high levels in the absence of signs of activation, which to our knowledge makes them the first naïve polyclonal T cells with cytotoxic features to have been described thus far. Notably, only T DC, and not T cells or DCs from naïve mice, expressed mRNA for granzyme A, a protease with unique properties such as being able to activate alternative death pathways [38] , [39] . A recent paper reports that a subset of murine immature DC deletes cognate CD8 + T cells through a mechanism mediated by perforin and granzyme A [40] . This raises the speculation that T DC might as well use their cytotoxic machinery to control an exacerbated immune response. The physiological role of T DC is currently being investigated by genetic approaches. Based on the fact that T DC combine features and functions of T cells and DCs, it is tempting to speculate that such duality might render T DC particularly responsive to infectious organisms, because they can bridge innate and adaptive traits. The contribution of T DC would be masked because, on TCR-mediated proliferation, T DC transiently lose DC markers, becoming indistinguishable from conventional T cells. However, as shown in responses to LCMV, antigen-experienced T DC re-acquire DC markers over time, suggesting long-term stability of their ‘mixed’ lineage. Infectious diseases are not the only context where T DC might have a role. To our knowledge, T DC are the first instance of an αβ-T cell that produces IL-12. Several reports show that tumor-specific T cells engineered to produce IL-12 are very effective in eliciting regression of, or even eradicating, melanomas [41] , [42] , [43] . One could envision that tumor-specific T DC might be effective in this setting because they produce IL-12 on stimulation, similar to innate APC. Thus, T DC , present in mice and humans, comprise a new and intriguing cell subset poised at the intersection of innate and adaptive immunity. Mice C57BL/6 (B6) and athymic nude mice were obtained from the NCI-Frederick Animal Facility. FLT3L-deficient mice were generated by Immunex as described [16] and purchased from Taconic. CD11c-Cre, CD11c-Cre-EGFP, ROSA26 flox STOP flox YFP, OTII TCR Tg, AND TCR Tg, and B6 mice-bearing CD45.1 or Thy-1.1 congenic markers were obtained from The Jackson Laboratory. Rosa26-CD11c-cre-YFP mice were obtained by breeding ROSA26 flox STOP flox YFP to CD11c-Cre mice. Thpok-GFP, Thpok −/− and P14 TCR Tg in B6 background mice were a kind gift of Dr Rémy Bosselut (NCI). The Animal Care and Use Committee of the National Cancer Institute approved all animal experimental procedures. Cells and reagents Purified or fluorochrome-conjugated antibodies to murine and human cell surface markers and cytokines were purchased from BD Biosciences or eBioscience. LCMV Armstrong strain was a gift from Dr Rafi Ahmed (Emory University School of Medicine). The H-2D b /LCMV gp33–41 (KAVYNFATC) tetramer labeled with allophycocyanin was obtained from the NIH Tetramer Core Facility at Emory University. LPS, brefeldin A and OVA were purchased from Sigma Aldrich, PolyI:C and Pam3CSK4 obtained from Invivogen, OVA 323–339 peptide obtained from Genscript, carboxyfluorescein diacetate succinimidyl ester obtained from Invitrogen and recombinant IL-2 and IFN-γ obtained from eBioscience. B16-FLT3L murine melanoma cells were a gift from Ulrich H. von Andrian (Harvard Medical School). B16-FLT3L-induced cell expansion in vivo B16-FLT3L cells were cultured in DMEM containing 10% fetal calf serum and antibiotics. Mice were injected subcutaneously with 10 6 B16-FLT3L cells and lymphoid cells were analyzed 10–13 days later. Cell preparation Thymus, spleen and lymph nodes were collected and total cell suspensions made by gently mashing the debris through 40-μM nylon mesh (BD Biosciences). Viable cells were counted by Trypan Blue exclusion, and the distribution of lymphoid populations in each organ was determined by cell surface staining and flow cytometry (LSRII, BD Biosciences). In some experiments, the indicated subsets underwent two or three rounds of sequential sorting to a purity of ≥99% (FACSAria I Cell Sorter obtained from BD Biosciences). Peripheral blood mononuclear cells from healthy donors were isolated from buffy coats of healthy donors using a Ficoll gradient (Ficoll-Paque PLUS obtained from GE Healthcare). Confocal microscopy Splenocytes were stained with antibodies to CD11c, MHC-II and TCRβ (H57), sorted to>99% purity and analyzed by confocal microscopy. Confocal images were sequentially acquired with Zeiss ZEN 2009 software on a Zeiss LSM 710 NLO Confocal system (Carl Zeiss Inc., Thornwood, NY, USA) with a Zeiss Observer Z1 inverted microscope and diode laser tuned to 405 nm, a 25-mW Argon visible laser tuned to 488 nm and a HeNe laser tuned to 633 nm. A 63X Plan-Apochromat 1.4 NA oil immersion objective was used and digital images were 512 × 512 pixels with 0.264-mm pixel size. Emission signals after sequential excitation of eFluor450, FITC and APC by the 405-nm, 488-nm or 633-nm laser lines were collected with a BP 419–485-nm filter, BP 495–534-nm filter and BP 650–710-nm filter, respectively, using individual photomultipliers. Cell culture and stimulation Cultures were performed with RPMI 1640 (Gibco) supplemented with 10% heat-inactivated fetal calf serum, glutamine, β-mercaptoethanol and antibiotics. Murine splenocytes or human peripheral blood mononuclear cells were stimulated with TLR agonists or with soluble anti-CD3ε (2C11) at the indicated concentrations. Activation markers were detected by surface staining 18–24 h later. In some experiments, brefeldin A (Sigma Aldrich) was added at a concentration of 10 μg ml −1 2 h after stimulation and after another 16–24 h cells were fixed and permeabilized (BD Cytofix/Cytoperm and Perm/Wash Buffer kit) and stained for IL-12. In some proliferation experiments, double-sorted cells were stimulated with soluble anti-CD3 (1 μg ml −1 ) and at day 3 the cultures were supplemented with IL-2 (20 U ml −1 ) for 5 more days. When indicated, sorted cells were labeled with carboxyfluorescein diacetate succinimidyl ester (0.5 μM) and stimulated with OVA peptide 323–339 or whole protein at the indicated concentrations. Adoptive transfers and LCMV infection P14 TCR Tg T cells from CD45.1 + mice or P14 TCR Tg T DC from Thy1.1 + mice were sorted, mixed 1:1 (5,000 cells total) and injected intravenous into B6 recipients. The day after adoptive transfer, mice were infected intraperitoneal with 2 × 10 5 plaque-forming units of LCMV Armstrong strain, and spleen and lymph node cells were analyzed 8 days later. In other experiments, endogenous responses to LCMV were determined by infecting B6 mice with LCMV Armstrong strain and analyzed 2 months later. Microarray analysis and RT–PCR Total RNA was isolated with the RNeasy Micro kit (Qiagen) from 1,000 to 4,000 cells that were double or triple sorted from B6 splenocytes. Microarray gene expression was performed by the Laboratory of Molecular Technology (NCI), with Affymetrix 430 2.0 GeneChip technology after RNA was amplified with a NuGEN WT-Ovation kit (Nugen). Microarray data analysis was performed with Partek Genomics Suite 6.6 (St Louis, MO, USA). One-way analysis of variance was applied to three samples with paired comparisons between samples (T DC versus T cells, T DC versus DCs and DCs versus T cells). For Ciita detection by RT–PCR, cDNA was synthesized using the SuperScriptTM II RT kit (Invitrogen) and RT–PCR was performed with Ciita primers (5′-CCAAAGGATGTGGAAGACCT-3′ and 5′-AGCTTCTTAAGGTCCCGGAT-3′) and Hprt primers (5′-AAACAATGCAAACTTTGCTTTCC-3′ and 5′-TCCTTTTCACCAGCAAGCTTG-3′). For the other genes SuperScript III One-Step RT–PCR System with Platinum Taq High Fidelity kit (Invitrogen) was used with gene-specific primers to retro-transcribe and amplify trancripts in one step. We used the following primer pairs: Eomes (5′-TCGTGGAAGTGACAGAGGAC-3′ and 5′-AGCTGGGTGATATCCGTGTT-3′), Gzma (5′-AGGCTGTGAAAGAATCATTGGAG-3′ and 5′-ATCCTGCTACTCGGCATCTGGTTC-3′), Gzmb (5′-ACTTTCGATCAAGGATCAGCA-3′ and 5′-ACTGTCAGCTCAACCTCTTGT-3′), Prf1 (5′-CAAGCAGAAGCACAAGTTCGT-3′ and 5′-GTGATAAAGTGCGTGCCATA-3′), Actb (5′-GTGGGCCGCCCTAGGCACC-3′ and 5′-TCTTTGATGTCACGCACGAT-3′), Sfpi1 (5′-TCCATCGGATGACTTGGTTA-3′ and 5′-AGGAAACCTGGTGACTGAGG-3′), Zbtb46 (5′-CCACTCACTGTCTCTGAACGA-3′ and 5′-CTTCTTGTCCTTGCTGTGGA-3′). How to cite this article: Kuka M. et al. Identification and characterization of polyclonal αβ-T cells with dendritic cell properties. Nat. Commun. 3:1223 doi: 10.1038/ncomms2223 (2012).